Migration of growth factor-stimulated epithelial and endothelial cells depends on EGFR transactivation by ADAM17 The fibroblast growth factor receptor 2-IIIb (FGFR2b) and the vascular endothelial growth factor receptor 2 (VEGFR2) are tyrosine kinases that can promote cell migration and proliferation and have important roles in embryonic development and cancer. Here we show that FGF7/FGFR2b-dependent activation of epidermal growth factor receptor (EGFR)/ERK1/2 signalling and cell migration in epithelial cells require stimulation of the membrane-anchored metalloproteinase ADAM17 and release of heparin-binding epidermal growth factor (HB-EGF). Moreover, VEGF-A/VEGFR2-induced migration of human umbilical vein endothelial cells also depends on EGFR/ERK1/2 signalling and shedding of the ADAM17 substrate HB-EGF. The pathway used by the FGF7/FGFR2b signalling axis to stimulate shedding of substrates of ADAM17, including ligands of the EGFR, involves Src, p38 mitogen-activated protein-kinase and PI3K, but does not require the cytoplasmic domain of ADAM17. Based on these findings, ADAM17 emerges as a central component in a triple membrane-spanning pathway between FGFR2b or VEGFR2 and EGFR/ERK1/2 that is required for cell migration in keratinocytes and presumably also in endothelial cells. Activation of the fibroblast growth factor receptor 2-IIIb (FGFR2b) by the fibroblast growth factor 7 (FGF7), also referred to as keratinocyte growth factor, is known to stimulate phosphorylation of the extracellular signal-regulated kinases ERK1/2 and to regulate the proliferation and migration of epithelial cells [1] , [2] , [3] , yet much remains to be learned about the underlying mechanism. Previous studies have shown that the cell surface metalloproteinase ADAM17 (a disintegrin and metalloproteinase 17) responds to stimulation by tyrosine kinases such as the vascular endothelial growth factor receptor 2 (VEGFR2) or G-protein coupled receptors, resulting in the release of ligands of the epidermal growth factor receptor (EGFR) and activation of ERK1/2 signalling [4] , [5] , [6] , [7] . ADAM17 has also emerged as a crucial physiological regulator of EGFR signalling during development, mainly because mice lacking ADAM17 resemble mice lacking the EGFR [8] , [9] or certain EGFR-ligands. Specifically, Adam17−/− mice have open eyes at birth (also seen in Tgfα−/− and hb-egf−/− mice [10] , [11] , [12] ), defects in cardiovascular morphogenesis with thickened and misshapen heart valves (also found in hb-egf−/− mice and in animals with a knock-in mutation in the cleavage site of heparin-binding epidermal growth factor-like growth factor (HB-EGF) [13] , [14] , [15] , [16] , [17] ), and defects in branching morphogenesis in the developing mammary gland (also observed in mice lacking amphiregulin [18] ). Thus, EGFR signalling is impaired in Adam17−/− mice, most likely because the soluble active forms of these EGFR-ligands are not generated at sufficient levels to stimulate EGFR when ADAM17 is deleted. The main goal of the current study was to evaluate what role, if any, ADAM17 has in the activation of EGFR/ERK1/2 in keratinocytes and in promoting their migration in response to FGF7/FGFR2b signalling [19] , [20] . In addition, as ADAM17 is known to be required for cross talk between the VEGFR2 and ERK1/2 in human umbilical vein endothelial cells (HUVECs) [4] , we were interested in determining the functional consequences of this cross talk, and therefore tested whether ADAM17 is required for the migration of HUVECs in response to activation of VEGF-A/VEGFR2 signalling. Our results uncovered a crucial role for ADAM17 in the FGF7/FGFR2b-dependent stimulation of the EGFR/ERK1/2 signalling pathway and of cell migration in primary human and mouse keratincytes as well as in HaCaTs, a human keratinocyte cell line. Moreover, we found that the VEGF-A-stimulated migration of HUVECs also depends on activation of a metalloproteinase and of the EGFR/ERK1/2 signalling axis. Our results suggest that ADAM17 is responsible for mediating the transactivation of the EGFR/ERK1/2 signalling pathway by two distinct receptor tyrosine kinases, FGFR2b and VEGFR2. Stimulation of ERK1/2 by FGFR2b requires a metalloproteinase To determine whether FGFR2b-dependent phosphorylation of ERK1/2 in keratinocytes requires activation of a metalloproteinase, we tested how the hydroxamate metalloproteinase inhibitor marimastat (MM) affects ERK1/2 phosphorylation at different time points after addition of FGF7 to primary human keratinocytes ( Fig. 1a,b ) or HaCaT cells, a human keratinocyte cell line ( Fig. 1c,d ). Following addition of FGF7, ERK1/2 phosphorylation was observed within 5 min and persisted for at least 60 min in both cell types ( Fig. 1a,c shows representative western blots, and Fig. 1b,d shows densitometric quantification of three western blots for each cell type). Interestingly, the FGF7-dependent phosphorylation of ERK1/2 was completely prevented by MM in primary human keratinocytes and HaCaT cells, even as early as 5 min after addition of FGF7 ( Fig. 1a–d ). This suggested that FGFR2b stimulated ERK1/2 by the activation of a metalloproteinase, and not through an intracellular signalling pathway [21] . In this respect, FGFR2b/ERK1/2 cross talk in keratinocytes differs significantly from the stimulation of ERK1/2 by VEGF-A/VEGFR2 in HUVECs, which consists of an early component that is not sensitive to MM, and a late component that is sensitive to MM ( Fig. 1e,f ; see also ref. 4 ). Thus, a major distinction between the stimulation of ERK1/2 by the tyrosine kinases FGFR2b and VEGFR2 is that VEGF-A/VEGFR2 can initially activate ERK1/2 via cross talk that is insensitive to metalloproteinase inhibition and therefore most likely intracellular, whereas FGFR2b apparently lacks the ability to stimulate ERK1/2 without the involvement of a metalloproteinase, at least in primary human keratinocytes and HaCaT cells (similar results were obtained with primary murine keratinocytes, see below). The activation of ERK1/2 by the tyrosine kinase receptor FGFR2b thus resembles the cross talk between several G-protein coupled receptors and ERK1/2, which also depends entirely on activation of metalloproteinases [7] , [22] . To corroborate this point, we treated mouse embryonic fibroblasts (mEFs) with thrombin to stimulate the G-protein coupled protease-activated receptor 1 (PAR1), which has previously been shown to activate ERK1/2 via stimulation of a metalloproteinase and EGFR [23] . We found a very similar time course and MM-sensitivity of ERK1/2 activation as we had observed in primary human keratinocytes or HaCaT cells treated with FGF7 ( Fig. 1g,h ). Thus, the FGF7/FGFR2b-dependent activation of ERK1/2 between 5 and 60 min after addition of FGF7 appears to rely predominantly, if not entirely, on a metalloproteinase. 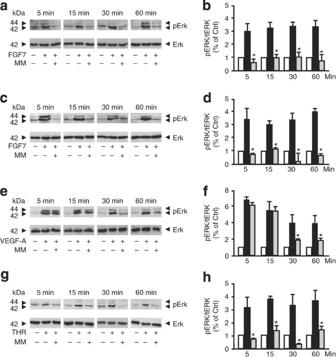Figure 1: Metalloproteinase-dependent cross talk between FGFR2b or the VEGFR2 and EGFR/ERK-signalling. A time course of ERK1/2 phosphorylation is shown for primary human keratinocytes (a,b) or HaCaT cells (c,d) treated with or without 20 ng ml−1FGF7; for HUVECs treated with or without 25 ng ml−1VEGF-A (e,f) or for mEFs treated in the presence or absence of 2 U ml−1thrombin (THR) (g,h), in each case with or without addition of 5 μM marimastat (MM) to the treated sample, as indicated. Representative western blot analyses of ERK1/2 phosphorylation at different time points are shown in (a,c,e,g), with an immunoblot of total ERK1/2 included as loading control, and the results of a densitometric quantification of ERK1/2 phosphorylation relative to total ERK are in (b,d,f,h). An asterisk indicates a significant decrease in ERK1/2 phosphorylation in the stimulated sample in the presence of 5 μM MM compared with in the absence of MM. White bars: unstimulated cells, black bars: stimulated cells, grey bars: stimulated cells in the presence of MM.n=3 for all densitometric quantifications; ± s.e.m; Student'st-test *P≤0.05. Figure 1: Metalloproteinase-dependent cross talk between FGFR2b or the VEGFR2 and EGFR/ERK-signalling. A time course of ERK1/2 phosphorylation is shown for primary human keratinocytes ( a , b ) or HaCaT cells ( c , d ) treated with or without 20 ng ml −1 FGF7; for HUVECs treated with or without 25 ng ml −1 VEGF-A ( e , f ) or for mEFs treated in the presence or absence of 2 U ml −1 thrombin (THR) ( g , h ), in each case with or without addition of 5 μM marimastat (MM) to the treated sample, as indicated. Representative western blot analyses of ERK1/2 phosphorylation at different time points are shown in ( a , c , e , g ), with an immunoblot of total ERK1/2 included as loading control, and the results of a densitometric quantification of ERK1/2 phosphorylation relative to total ERK are in ( b , d , f , h ). An asterisk indicates a significant decrease in ERK1/2 phosphorylation in the stimulated sample in the presence of 5 μM MM compared with in the absence of MM. White bars: unstimulated cells, black bars: stimulated cells, grey bars: stimulated cells in the presence of MM. n =3 for all densitometric quantifications; ± s.e.m; Student's t -test * P ≤0.05. Full size image FGFR2b and VEGFR2 stimulate shedding of HB-EGF We next tested whether activation of FGFR2b or VEGFR2 triggers the release of EGFR-ligands in stimulated primary human keratinocytes or HUVECs, respectively. Previous studies had demonstrated that activation of the VEGFR2 by VEGF-A stimulates ADAM17 to release ligands of EGFR in a variety of different cell types, but these studies relied on transfected alkaline phosphatase (AP)-tagged EGFR-ligands as a readout [4] . We therefore decided to use conditioned supernatants from FGF7-treated primary human keratinocytes to stimulate A431 cells (an EGFR-overexpressing cell line [24] ) to provide evidence for the release of endogenous EGFR ligands from human keratinocytes. When the conditioned supernatants of human keratinocytes that had been stimulated with FGF7 for 5–60 min were applied to A431 cells, we observed an increase in ERK1/2 phosphorylation in the A431 cells, with the supernatant of unstimulated human keratinocytes serving as control ( Fig. 2a,b ). In all cases, supernatants of FGF7-stimulated human keratinocytes conditioned in the presence of MM elicited only background levels of ERK1/2 phosphorylation in the A431 cells (note that all conditioned supernatants were adjusted to the same concentration of MM before addition to A431 cells to rule out that this metalloproteinase inhibitor affects ERK1/2 activation in A431 cells). Moreover, stimulation of ERK1/2 phosphorylation in A431 by conditioned supernatants of human keratinocytes treated with FGF7 could be reduced by the mutant diphtheria toxin CRM197, which selectively inactivates the human form of HB-EGF [25] , by the EGFR-kinase inhibitor AG1478 and the EGFR-function blocking antibody Cetuximab ( Fig. 2c,d ), further corroborating that activation of the EGFR by the conditioned supernatants is crucial for ERK1/2 phosphorylation in A431 cells. Identical experiments with conditioned supernatants of VEGF-A-treated HUVECs showed a comparable metalloproteinase-dependent activation of ERK1/2 in A431 cells, with activation of ERK1/2 elicited by supernatants of HUVECs that had been treated with VEGF-A for as little as 5 min ( Fig. 2e,f ). The ERK1/2 phosphorylation in A431 cells triggered by supernatants of VEGF-A-treated HUVECs could also be blocked by CRM197, AG1478 and Cetuximab ( Fig. 2g,h ). Finally, we found that treatment of A431 cells with VEGF-A or FGF7 did not stimulate ERK1/2 phosphorylation, ruling out that the activation of ERK1/2 in these cells was stimulated directly by the VEGF-A or FGF7 present in the conditioned supernatants ( Fig. 2i,j ). 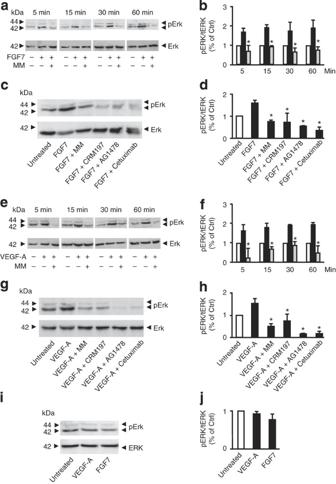Figure 2: Conditioned supernatants from FGF7-stimulated human primary keratinocytes or VEGF-A-stimulated HUVECs activate ERK1/2. Western blot of ERK1/2 phosphorylation in A431 cells treated with conditioned supernatants of primary human keratinocytes that had been incubated for 5–60 min in the presence or absence of 20 ng ml−1FGF7, with or without 5 μM MM (a) and densitometric quantification of ERK1/2 phosphorylation relative to total ERK (b, white bar: no FGF; black bar: FGF7; grey bar: FGF7 plus marimastat). Representative immunoblot of ERK1/2 phosphorylation in A431 cells treated for 10 min with conditioned supernatants of primary human keratinocytes that were incubated for 10 min with control medium, or with medium containing FGF7, or FGF7 and 5 μM MM, or 10 μg ml−1of the mutant diphtheria toxin CRM197, or 1 μM of the EGFR-kinase inhibitor AG1478, or 10 μg ml−1the EGFR-function blocking antibody Cetuximab (C225), respectively (c), and densitometric quantification (d). Representative immunoblot of ERK1/2 phosphorylation elicited in A431 cells by a 10-min treatment with conditioned supernatants of HUVECs that were cultured in the presence or absence of 25 ng ml−1VEGF-A, or VEGF-A and 5 μM MM for various amounts of time, as indicated (e), and densitometric quantification (f, white bar: no VEGF; black bar: VEGF; grey bar: VEGF plus marimastat). Western blot of ERK1/2 phosphorylation in A431 cells treated for 10 min with conditioned supernatants from HUVECs cultured for 10 min with or without VEGF-A, or with VEGF-A and MM, CRM197, AG1478, or Cetuximab (g), and densitometric quantification (h). Representative immunoblot of ERK1/2 phosphorylation in A431 cells treated with VEGF-A or FGF7 (i) and densitometric quantification of three separate blots (j). An asterisk indicates significantly decreased ERK1/2 phosphorylation in the stimulated sample in the presence of various inhibitors compared with the absence of those inhibitors, as indicated.n=3 for all densitometric quantifications; ±s.e.m; Student'st-test *P≤0.05. Figure 2: Conditioned supernatants from FGF7-stimulated human primary keratinocytes or VEGF-A-stimulated HUVECs activate ERK1/2. Western blot of ERK1/2 phosphorylation in A431 cells treated with conditioned supernatants of primary human keratinocytes that had been incubated for 5–60 min in the presence or absence of 20 ng ml −1 FGF7, with or without 5 μM MM ( a ) and densitometric quantification of ERK1/2 phosphorylation relative to total ERK ( b , white bar: no FGF; black bar: FGF7; grey bar: FGF7 plus marimastat). Representative immunoblot of ERK1/2 phosphorylation in A431 cells treated for 10 min with conditioned supernatants of primary human keratinocytes that were incubated for 10 min with control medium, or with medium containing FGF7, or FGF7 and 5 μM MM, or 10 μg ml −1 of the mutant diphtheria toxin CRM197, or 1 μM of the EGFR-kinase inhibitor AG1478, or 10 μg ml −1 the EGFR-function blocking antibody Cetuximab (C225), respectively ( c ), and densitometric quantification ( d ). Representative immunoblot of ERK1/2 phosphorylation elicited in A431 cells by a 10-min treatment with conditioned supernatants of HUVECs that were cultured in the presence or absence of 25 ng ml −1 VEGF-A, or VEGF-A and 5 μM MM for various amounts of time, as indicated ( e ), and densitometric quantification ( f , white bar: no VEGF; black bar: VEGF; grey bar: VEGF plus marimastat). Western blot of ERK1/2 phosphorylation in A431 cells treated for 10 min with conditioned supernatants from HUVECs cultured for 10 min with or without VEGF-A, or with VEGF-A and MM, CRM197, AG1478, or Cetuximab ( g ), and densitometric quantification ( h ). Representative immunoblot of ERK1/2 phosphorylation in A431 cells treated with VEGF-A or FGF7 ( i ) and densitometric quantification of three separate blots ( j ). An asterisk indicates significantly decreased ERK1/2 phosphorylation in the stimulated sample in the presence of various inhibitors compared with the absence of those inhibitors, as indicated. n =3 for all densitometric quantifications; ±s.e.m; Student's t -test * P ≤0.05. Full size image FGF7-stimulated keratinocyte migration requires ADAM17 To assess the functional relevance of metalloproteinase-dependent EGFR/ERK1/2 signalling in FGF7-stimulated keratinocytes, we performed in vitro scratch wound healing assays with HaCaT cells ( Fig. 3 ) or primary human keratinocytes ( Supplementary Fig. S1 ) in the presence or absence of MM or Cetuximab. Untreated HaCaT cells or primary human keratinocytes did not repair scratch wounds after 12 h, but treatment with FGF7 led to complete closure of the wound in 12 h ( Fig. 3a , Supplementary Fig. S1a ). FGF7-stimulated migration of HaCaT cells and primary human keratinocytes could be blocked by MM and Cetuximab ( Fig. 3a , Supplementary Fig. S1a ). The inhibition of FGF7-dependent cell migration by MM could be rescued by addition of human HB-EGF ( Fig. 3a , Supplementary Fig. S1a ), which is known to require processing by the membrane-anchored metalloproteinase ADAM17 (a disintegrin and metalloproteinase 17) [13] , [14] , [26] , [27] , [28] . However, HB-EGF did not rescue the inhibition by Cetuximab, as this blocks binding of HB-EGF to the EGFR ( Fig. 3a , Supplementary Fig. S1a , a quantification of the results of three separate experiments is shown in Fig. 3b and Supplementary Fig. S1b , respectively). A western blot analysis of similarly treated cultures demonstrated that addition of FGF7 increased phosphorylation of EGFR ( Fig. 3c,d ) and ERK1/2 in HaCaT cells ( Fig. 3e,f ) and of ERK1/2 in primary human keratinocytes ( Supplementary Fig. S1c,d ), which could be prevented in both cell types if FGF7 was applied together with MM or Cetuximab. Moreover, EGFR and ERK1/2 phosphorylation was strongly stimulated by adding HB-EGF to cultures treated with FGF7 and MM, whereas HB-EGF did not activate EGFR or ERK1/2 in the presence of Cetuximab ( Fig. 3c–f , only ERK1/2 phosphorylation of primary human keratinocytes is shown in Supplementary Fig. S1c,d ). Neither MM nor Cetuximab had any detectable effect on the phosphorylation of the FGFR2b target FRS2 in HaCaTs, arguing against direct effects of MM or Cetuximab on the activation of FGFR2b by FGF7 ( Fig. 3g,h ). 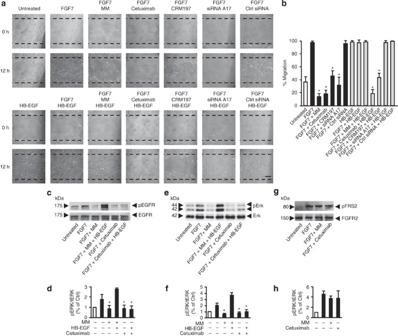Figure 3: FGF7-stimulated epithelial cell migration depends on ADAM17 and EGFR. (a) HaCaT cells were treated with or without FGF7 (50 ng ml−1) or HB-EGF (50 ng ml−1) in the presence or absence of MM (5 μM), Cetuximab (10 μg ml−1), CRM197 (10 μg ml−1), siRNA against ADAM17 or control siRNA (50 nM). A cell-free area was introduced with a pipette tip, and micrographs were taken at 0 and 12 h after scratch wounding. One representative of three independent experiments is shown. Scale bar, 100 μm. (b) Quantification of the results of three separatein vitroscratch wound assays. Asterisks (*) indicate a significant decrease compared with FGF7-treated samples. Western blot analysis of the effect of MM and Cetuximab on the FGF7 stimulated EGFR phosphorylation in HaCaT cells (c) and densitometric quantification (d). Cells were pre-incubated for 15 min with MM (5 μM) or Cetuximab (10 μg ml−1) and then stimulated with FGF7 or FGF7/HB-EGF. (e,f) Representative immunoblot of ERK1/2 phosphorylation in FGF7-stimulated HaCaT cells in the presence or absence of MM or Cetuximab (e), and quantification of ERK1/2 phosphorylation (f). Western blot of lysates of FGF7-stimulated HaCaT cells show that neither MM nor Cetuximab significantly affect the stimulation of the FGFR2b target FRS2 (g) and densitometric quantification (h). White bars: no stimulation, black bars: stimulation with FGF7. An asterisk indicates a significant decrease in ERK1/2 phosphorylation in the stimulated sample in the presence of various inhibitors compared with the absence of inhibitors.n=3 for all densitometric quantifications; ±s.e.m; Student'st-test *P≤0.05. Figure 3: FGF7-stimulated epithelial cell migration depends on ADAM17 and EGFR. ( a ) HaCaT cells were treated with or without FGF7 (50 ng ml −1 ) or HB-EGF (50 ng ml −1 ) in the presence or absence of MM (5 μM), Cetuximab (10 μg ml −1 ), CRM197 (10 μg ml −1 ), siRNA against ADAM17 or control siRNA (50 nM). A cell-free area was introduced with a pipette tip, and micrographs were taken at 0 and 12 h after scratch wounding. One representative of three independent experiments is shown. Scale bar, 100 μm. ( b ) Quantification of the results of three separate in vitro scratch wound assays. Asterisks (*) indicate a significant decrease compared with FGF7-treated samples. Western blot analysis of the effect of MM and Cetuximab on the FGF7 stimulated EGFR phosphorylation in HaCaT cells ( c ) and densitometric quantification ( d ). Cells were pre-incubated for 15 min with MM (5 μM) or Cetuximab (10 μg ml −1 ) and then stimulated with FGF7 or FGF7/HB-EGF. ( e , f ) Representative immunoblot of ERK1/2 phosphorylation in FGF7-stimulated HaCaT cells in the presence or absence of MM or Cetuximab ( e ), and quantification of ERK1/2 phosphorylation ( f ). Western blot of lysates of FGF7-stimulated HaCaT cells show that neither MM nor Cetuximab significantly affect the stimulation of the FGFR2b target FRS2 ( g ) and densitometric quantification ( h ). White bars: no stimulation, black bars: stimulation with FGF7. An asterisk indicates a significant decrease in ERK1/2 phosphorylation in the stimulated sample in the presence of various inhibitors compared with the absence of inhibitors. n =3 for all densitometric quantifications; ±s.e.m; Student's t -test * P ≤0.05. Full size image Additional scratch wound healing experiments performed with HaCaT cells in the presence of FGF7 showed that CRM197 also significantly decreased cell migration ( Fig. 3a ). The requirement of HB-EGF for FGF7-stimulated migration of HaCaT cells raised the possibility that the HB-EGF sheddase ADAM17 (refs 13 , 14 , 26 , 27 , 28 ) is a critical intermediate in the signalling pathway between the FGF7/FGFR2b and EGFR/ERK1/2. To test this possibility, HaCaT cells were treated with anti-ADAM17 short interfering RNA (siRNA), which blocked FGF7-stimulated cell migration, whereas treatment with control siRNA did not ( Fig. 3a ). HB-EGF could rescue the defect in cell migration caused by treatment of FGF7-stimulated cells with ADAM17 siRNA, but could not rescue migration of cells treated with CRM197 ( Fig. 3a ). A quantification of the scratch wound healing results described above in three independent experiments is shown in Figure 3b . A western blot analysis of HaCaT cells confirmed that FGF7-stimulated ERK1/2 phosphorylation was blocked by CRM197 ( Supplementary Fig. S2a ) by siRNA against ADAM17, but not by control siRNA ( Supplementary Fig. S2b ). An immunoblot for ADAM17 confirmed that the siRNA treatment strongly reduced expression of ADAM17, whereas treatment with control siRNA had no effect compared with untreated cells ( Supplementary Fig. S2c ). Finally, we corroborated that Cetuximab did not block the FGF7-stimulated activation of ADAM17 in HaCaT cells, using shedding of transforming growth factor-α (TGFα) as a readout ( Supplementary Fig. S2d ). Conditional inactivation of ADAM17 in murine keratinocytes As a next step, we wished to provide genetic evidence for a role of ADAM17 in FGF7-stimulated keratinocyte migration. For this purpose, primary keratinocytes were isolated from Tamoxifen-inducible conditional knockout mice for ADAM17 ( Adam17flox/flox/CAG-Cre ) or control mice that carried two floxed alleles of ADAM17, but not the Tamoxifen inducible Cre-driver ( Adam17flox/flox , see Methods ). In scratch wound healing assays, treatment with FGF7 for 18 h increased the migration of control primary keratinocytes from Adam17flox/flox mice, regardless of whether they had been treated with Tamoxifen ( Fig. 4a ). However, migration of Tamoxifen-treated keratinocytes from Adam17flox/flox/CAG-Cre mice was only weakly stimulated by FGF7, whereas the response of untreated Adam17flox/flox/CAG-Cre keratinocytes was comparable with that of control Adam17flox/flox keratinocytes ( Fig. 4b ). Cell migration of Tamoxifen-treated keratinocytes from Adam17flox/flox/CAG-Cre mice could be stimulated by addition of HB-EGF ( Fig. 4b ; a quantification of the results from three separate experiments is shown in Fig. 4c–f ). A western blot analysis confirmed that Tamoxifen treatment efficiently reduced the expression of ADAM17 in keratinocytes from Adam17flox/flox/CAG-Cre mice, whereas it had no effect on controls from Adam17flox/flox mice ( Fig. 4g ). In cross talk experiments like those shown in Figure 1 , FGF7 treatment activated ERK1/2 in a MM-sensitive manner in Adam17flox/flox controls, and this response was not significantly affected by pretreatment with Tamoxifen ( Fig. 4h,i ). However, in Adam17flox/flox/CAG-Cre keratinocytes, ERK1/2 phosphorylation in response to FGF7 was only seen in untreated cells, but not in cells that were pretreated with Tamoxifen to induce excision of ADAM17 ( Fig. 4j,k ). Addition of HB-EGF resulted in ERK1/2 phosphorylation in Adam17flox/flox control cells and Adam17flox/flox/CAG-Cre cells incubated with FGF7 and MM, regardless of whether they had been pretreated with Tamoxifen ( Fig. 4h–k ), demonstrating that deletion of ADAM17 did not affect the ability of EGFR to respond to HB-EGF. Finally, the FGF7-stimulated proliferation of Tamoxifen-treated or untreated Adam17flox/flox control keratinocytes over a time course of 72 h was comparable ( Fig. 4l,m ), whereas the FGF7-stimulated proliferation of Tamoxifen-treated primary mouse keratinocytes from Adam17flox/flox/CAG-Cre mice was strongly reduced compared with that of otherwise identical cells that were not treated with Tamoxifen ( Fig. 4n,o ). The proliferation of Tamoxifen-treated Adam17flox/flox/CAG-Cre keratinocytes could be stimulated by HB-EGF, demonstrating that EGFR-dependent proliferation was not affected ( Fig. 4o ). 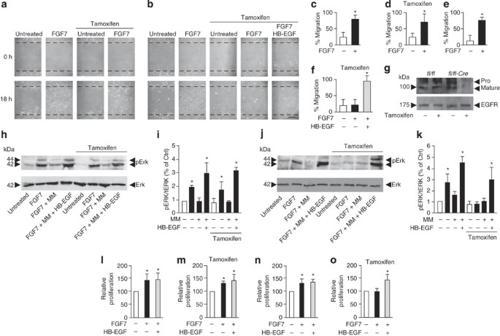Figure 4: Tamoxifen-induced inactivation of ADAM17 reduces FGF7-stimulated keratinocyte migration and proliferation. Primary keratinocytes from mice with two floxedAdam17alleles, but no Tamoxifen-inducible Cre (Adam17flox/flox) (a) or from Tamoxifen-inducible conditional knockout mice for ADAM17 (Adam17flox/flox/CAG-Cre)(b) were treated with 1 μM Tamoxifen for 48 h and then cultured in keratinocyte growth medium for 12 h. Subsequently a scratch wound was introduced and the cultures were treated with or without FGF7 (50 ng ml−1) or HB-EGF (50 ng ml−1). Micrographs were taken at 0 and 18 h after scratch wounding. Scale bar, 100 μm. Quantification of three separatein vitroscratch wound assays with untreated primaryAdam17flox/floxkeratinocytes (c), Tamoxifen-treated primaryAdam17flox/floxkeratinocytes (d), untreated primaryAdam17flox/flox/CAG-Crekeratinocytes (e) or Tamoxifen-treated primaryAdam17flox/flox/CAG-Crekeratinocytes (f). Asterisks (*) indicate a significant increase in cell migration in the treated samples compared with untreated controls. The cells were collected after 60 h and analysed for ADAM17 expression by western blot (g). (h–k) ERK1/2 phosphorylation in primary keratinocytes fromAdam17flox/floxcontrol mice (h,i) orAdam17flox/flox/CAG-Cremice (j,k) treated with or without Tamoxifen for 48 h. Representative western blots are depicted inhandj, and the corresponding densitometric quantifications of ERK1/2 phosphorylation in western blots of three separate experiments are shown iniandk. After 6 h recovery from Tamoxifen treatment, the cells were incubated with or without FGF7 (20 ng ml−1) or HB-EGF (50 ng ml−1) in the presence or absence of MM (5 μM). Total ERK1/2 served as loading control. (l–o) Proliferation of primaryAdam17flox/floxkeratinocytes (l), Tamoxifen-treated primaryAdam17flox/floxkeratinocytes (m), primaryAdam17flox/flox/CAG-Crekeratinocytes (n) or Tamoxifen-treated primaryAdam17flox/flox/CAG-Crekeratinocytes (o) incubated with or without FGF7 (20 ng ml−1) or HB-EGF (50 ng ml−1), as indicated. White bars: no stimulation, black bars: stimulation with FGF7, grey bars: stimulation with FGF7 and HB-EGF. An asterisk indicates a significant decrease in ERK1/2 phosphorylation in the stimulated sample with inhibitors compared with the sample without inhibitors.n=3; ±s.e.m; Student'st-test *P≤0.05. Figure 4: Tamoxifen-induced inactivation of ADAM17 reduces FGF7-stimulated keratinocyte migration and proliferation. Primary keratinocytes from mice with two floxed Adam17 alleles, but no Tamoxifen-inducible Cre ( Adam17flox/flox ) ( a ) or from Tamoxifen-inducible conditional knockout mice for ADAM17 ( Adam17flox/flox/CAG-Cre) ( b ) were treated with 1 μM Tamoxifen for 48 h and then cultured in keratinocyte growth medium for 12 h. Subsequently a scratch wound was introduced and the cultures were treated with or without FGF7 (50 ng ml −1 ) or HB-EGF (50 ng ml −1 ). Micrographs were taken at 0 and 18 h after scratch wounding. Scale bar, 100 μm. Quantification of three separate in vitro scratch wound assays with untreated primary Adam17flox/flox keratinocytes ( c ), Tamoxifen-treated primary Adam17flox/flox keratinocytes ( d ), untreated primary Adam17flox/flox/CAG-Cre keratinocytes ( e ) or Tamoxifen-treated primary Adam17flox/flox/CAG-Cre keratinocytes ( f ). Asterisks (*) indicate a significant increase in cell migration in the treated samples compared with untreated controls. The cells were collected after 60 h and analysed for ADAM17 expression by western blot ( g ). ( h – k ) ERK1/2 phosphorylation in primary keratinocytes from Adam17flox/flox control mice ( h , i ) or Adam17flox/flox/CAG-Cre mice ( j , k ) treated with or without Tamoxifen for 48 h. Representative western blots are depicted in h and j , and the corresponding densitometric quantifications of ERK1/2 phosphorylation in western blots of three separate experiments are shown in i and k . After 6 h recovery from Tamoxifen treatment, the cells were incubated with or without FGF7 (20 ng ml −1 ) or HB-EGF (50 ng ml −1 ) in the presence or absence of MM (5 μM). Total ERK1/2 served as loading control. ( l – o ) Proliferation of primary Adam17flox/flox keratinocytes ( l ), Tamoxifen-treated primary Adam17flox/flox keratinocytes ( m ), primary Adam17flox/flox/CAG-Cre keratinocytes ( n ) or Tamoxifen-treated primary Adam17flox/flox/CAG-Cre keratinocytes ( o ) incubated with or without FGF7 (20 ng ml −1 ) or HB-EGF (50 ng ml −1 ), as indicated. White bars: no stimulation, black bars: stimulation with FGF7, grey bars: stimulation with FGF7 and HB-EGF. An asterisk indicates a significant decrease in ERK1/2 phosphorylation in the stimulated sample with inhibitors compared with the sample without inhibitors. n =3; ±s.e.m; Student's t -test * P ≤0.05. Full size image VEGF-A-stimulated migration of HUVECs depends on HB-EGF When similar experiments were performed with HUVEC cells, a strong inhibition of VEGF-A-stimulated cell migration by treatment with MM for 12 h was observed, and this block in cell migration could be rescued by addition of HB-EGF ( Fig. 5a ). Pretreatment of HUVECs with Cetuximab, CRM197 or AG1478 also strongly reduced VEGF-A-stimulated migration. The inhibition of cell migration could be reversed by addition of EGF following CRM197 treatment (please note that CRM197 does not bind to EGF), whereas HB-EGF did not rescue the inhibition by Cetuximab or AG1478 ( Fig. 5a , a quantification of the results of three independent experiments is shown in Fig. 5b ). Western blot analysis of ERK1/2 phosphorylation in VEGF-A-stimulated HUVECs demonstrated that AG1478, Cetuximab and CRM197 blocked ERK1/2 phosphorylation as efficiently as MM ( Fig. 5c–h ). 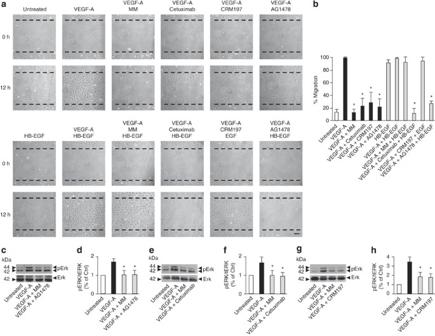Figure 5: VEGF-A-stimulated migration of HUVECs depends on a metalloproteinase and activation of EGFR. (a) Human umbilical vein endothelial cells (HUVECs) were treated with or without VEGF-A (25 ng ml−1) or HB-EGF (50 ng ml−1) in the presence or absence of 5 μM MM, 10 μg ml−1Cetuximab, 10 μg ml−1CRM197 or 1 μM AG1478. A scratch wound was introduced with a pipette tip, and micrographs of the same area on the tissue culture plate were taken at 0 and 12 h after wounding. VEGF-A-stimulated migration was blocked by MM, Cetuximab, CRM197 and AG1478. Addition of HB-EGF could rescue the migration of cells treated with VEGF-A and MM, and EGF could rescue migration of cells treated with VEGF-A and CRM197 (note that EGF was used in this sample because CRM197 inactivates human HB-EGF but not EGF25). One representative of three independent experiments is shown. Scale bar, 100 μm. (b) Quantification of the results of three separatein vitroscratch wound assays. (c–h) Western blot of phosphorylated ERK1/2 and total ERK1/2 in lysates of HUVECs treated with VEGF-A for 15 min in the presence or absence of MM or AG1478 (c), Cetuximab (e) or CRM197 (g). Quantification of the results in (c,e,g) is shown in (d,f,h), respectively. Asterisks (*) indicate a significant decrease compared with the VEGF-A- or HB-EGF-treated samples in the presence of any of the compounds listed above.n=3 for all densitometric quantifications; ±s.e.m; Student'st-test *P≤0.05. Figure 5: VEGF-A-stimulated migration of HUVECs depends on a metalloproteinase and activation of EGFR. ( a ) Human umbilical vein endothelial cells (HUVECs) were treated with or without VEGF-A (25 ng ml −1 ) or HB-EGF (50 ng ml −1 ) in the presence or absence of 5 μM MM, 10 μg ml −1 Cetuximab, 10 μg ml −1 CRM197 or 1 μM AG1478. A scratch wound was introduced with a pipette tip, and micrographs of the same area on the tissue culture plate were taken at 0 and 12 h after wounding. VEGF-A-stimulated migration was blocked by MM, Cetuximab, CRM197 and AG1478. Addition of HB-EGF could rescue the migration of cells treated with VEGF-A and MM, and EGF could rescue migration of cells treated with VEGF-A and CRM197 (note that EGF was used in this sample because CRM197 inactivates human HB-EGF but not EGF [25] ). One representative of three independent experiments is shown. Scale bar, 100 μm. ( b ) Quantification of the results of three separate in vitro scratch wound assays. ( c – h ) Western blot of phosphorylated ERK1/2 and total ERK1/2 in lysates of HUVECs treated with VEGF-A for 15 min in the presence or absence of MM or AG1478 ( c ), Cetuximab ( e ) or CRM197 ( g ). Quantification of the results in ( c , e , g ) is shown in ( d , f , h ), respectively. Asterisks (*) indicate a significant decrease compared with the VEGF-A- or HB-EGF-treated samples in the presence of any of the compounds listed above. n =3 for all densitometric quantifications; ±s.e.m; Student's t -test * P ≤0.05. Full size image ADAM17 is activated by FGFR2b To provide additional insights into the mechanism underlying the FGF7-stimulated release of EGFR-ligands, we evaluated the proteolytic release of AP-tagged HB-EGF, a substrate for ADAM17, from Cos-7 cells cotransfected with FGFR2b. We observed a significant dose-dependent increase in the shedding of HB-EGF from Cos-7 cells stimulated with 0.1–20 ng ml −1 FGF7 ( Fig. 6a ). These results further corroborate that the FGF7/FGFR2b signalling axis activates ADAM17. When similar experiments were performed with Cos-7 cells expressing the ADAM10-substrate betacellulin (BTC) [14] , no FGF7-stimulated increase in shedding of BTC was observed, even at the highest concentration of FGF7 (20 ng ml −1 , Fig. 6b ), indicating that ADAM10 is not activated by FGF7/FGFR2b signalling under these conditions. 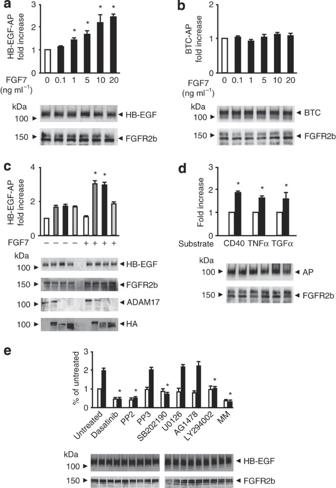Figure 6: FGF7/FGFR2b signalling activates ADAM17. (a) To measure activation of ADAM17 by FGF7/FGFR2b, Cos-7 cells were transfected with the alkaline phosphatase (AP)-tagged ADAM17-substrate HB-EGF14and FGFR2b, and stimulated with 0.1–20 ng ml−1FGF7. (b) To assess the response of ADAM10 to stimulation by FGF7/FGFR2b, similar experiments were performed with the AP-tagged ADAM10-substrate betacellulin (BTC)14. (c) Shedding of HB-EGF fromAdam17−/−cells expressing FGFR2b and inactive ADAM17E>A (white bar), wild-type ADAM17 (dark grey bar), ADAM17Δ-cyto lacking its cytoplasmic domain (black bar) or ADAM17-CD62L with the transmembrane domain of CD62L30(light grey bar), treated with or without FGF7. The western blots show controls for expression of FGFR2b, and of ADAM17E>A and ADAM17wt, detected with anti-cytoplasmic domain antibodies47and wild-type ADAM17, ADAM17Δ-cyto and ADAM17-CD62L, detected by western blot for an HA tag at the carboxy-terminus of these constructs. Please note that expression of ADAM17Δ-cyto is usually weaker than ADAM17wt, even though it can fully rescueAdam17−/−mEFs27,30,49. (d) Shedding of the ADAM17-substrates CD40, TNFα and TGFα from Cos-7 cells co-transfected with FGFR2b in the absence or presence of FGF7 (white and dark bars, respectively). (e) Effect of signalling inhibitors on HB-EGF shedding from FGF7-stimulated Cos-7 cells transfected with FGFR2b. Constitutive and FGF7-stimulated shedding (white and dark bars, respectively) was assessed either without further additions or in the presence of 10 μM of the Src-family kinase inhibitors Dasatinib or PP2, or the inactive PP2 analog PP3, the p38 MAP-kinase inhibitor SB202190 (10 μM), the MEK1/2 inhibitor U0126 (10 μM), the EGFR inhibitor AG1478 (1 μM), the PI3-kinase inhibitor LY294002 (10 μM) or MM (5 μM). Panelsa,b,dandeinclude controls to document comparable expression of alkaline phosphatase-tagged substrates and of FGFR2b. Ina,candd, an asterisk indicates significantly increased shedding in FGF7-treated cells compared with untreated controls. Ine, an asterisk indicates a significant decrease in FGF7-stimulated shedding in the presence of an inhibitor compared with cells treated with FGF7 only.n=3, ±s.e.m; Student'st-test *P≤0.05. Figure 6: FGF7/FGFR2b signalling activates ADAM17. ( a ) To measure activation of ADAM17 by FGF7/FGFR2b, Cos-7 cells were transfected with the alkaline phosphatase (AP)-tagged ADAM17-substrate HB-EGF [14] and FGFR2b, and stimulated with 0.1–20 ng ml −1 FGF7. ( b ) To assess the response of ADAM10 to stimulation by FGF7/FGFR2b, similar experiments were performed with the AP-tagged ADAM10-substrate betacellulin (BTC) [14] . ( c ) Shedding of HB-EGF from Adam17−/− cells expressing FGFR2b and inactive ADAM17E>A (white bar), wild-type ADAM17 (dark grey bar), ADAM17Δ-cyto lacking its cytoplasmic domain (black bar) or ADAM17-CD62L with the transmembrane domain of CD62L [30] (light grey bar), treated with or without FGF7. The western blots show controls for expression of FGFR2b, and of ADAM17E>A and ADAM17wt, detected with anti-cytoplasmic domain antibodies [47] and wild-type ADAM17, ADAM17Δ-cyto and ADAM17-CD62L, detected by western blot for an HA tag at the carboxy-terminus of these constructs. Please note that expression of ADAM17Δ-cyto is usually weaker than ADAM17wt, even though it can fully rescue Adam17−/− mEFs [27] , [30] , [49] . ( d ) Shedding of the ADAM17-substrates CD40, TNFα and TGFα from Cos-7 cells co-transfected with FGFR2b in the absence or presence of FGF7 (white and dark bars, respectively). ( e ) Effect of signalling inhibitors on HB-EGF shedding from FGF7-stimulated Cos-7 cells transfected with FGFR2b. Constitutive and FGF7-stimulated shedding (white and dark bars, respectively) was assessed either without further additions or in the presence of 10 μM of the Src-family kinase inhibitors Dasatinib or PP2, or the inactive PP2 analog PP3, the p38 MAP-kinase inhibitor SB202190 (10 μM), the MEK1/2 inhibitor U0126 (10 μM), the EGFR inhibitor AG1478 (1 μM), the PI3-kinase inhibitor LY294002 (10 μM) or MM (5 μM). Panels a , b , d and e include controls to document comparable expression of alkaline phosphatase-tagged substrates and of FGFR2b. In a , c and d , an asterisk indicates significantly increased shedding in FGF7-treated cells compared with untreated controls. In e , an asterisk indicates a significant decrease in FGF7-stimulated shedding in the presence of an inhibitor compared with cells treated with FGF7 only. n =3, ±s.e.m; Student's t -test * P ≤0.05. Full size image To further confirm that FGFR2b stimulates shedding of HB-EGF by activating ADAM17, we performed similar experiments in Adam17−/− mEFs. When Adam17−/− mEFs were cotransfected with FGFR2b, HB-EGF and an inactive form of ADAM17 containing an E to A point mutation in its catalytic site, FGF7 was unable to stimulate HB-EGF shedding ( Fig. 6c , white bars). When wild-type ADAM17 was cotransfected with FGFR2b and HB-EGF into Adam17−/− cells, this increased constitutive shedding and restored the FGF7-induced shedding of HB-EGF ( Fig. 6c , grey bars). A recent study has suggested that phosphorylation of the cytoplasmic domain of ADAM17 by mitogen-activated protein (MAP)-kinase is required for ADAM17-mediated ectodomain shedding [29] . However, a mutant ADAM17 lacking its cytoplasmic domain, and therefore all potential cytoplasmic phosphorylation sites, was able to rescue FGF7-stimulated shedding of HB-EGF equally well as wild-type ADAM17, arguing against a role of the cytoplasmic domain of ADAM17 in its activation by FGF7/FGFR2b ( Fig. 6c , black bars). On the other hand, when the transmembrane domain of ADAM17 was replaced with that of one of its substrates, CD62L, this prevented the response of ADAM17 to FGF7 ( Fig. 6c , light grey bars), as also previously described for other activators of ADAM17 (ref. 30 ). Finally, stimulation of Cos-7 cells with FGF7 increased shedding of three other ADAM17 substrates, CD40, TGFα and tumour-necrosis factor-α (TNFα; Fig. 6d ). Very similar findings were obtained when an essentially identical set of experiments was performed using TGFα as a substrate to monitor the activity of ADAM17 ( Supplementary Fig. S3a,b ). Taken together, these results demonstrate that FGF7/FGFR2b activates ADAM17, but not ADAM10. FGFR2b stimulates ADAM17 via a downstream signalling cascade To elucidate the signalling pathways involved in the FGF7/FGFR2b-dependent activation of ADAM17, we tested how various inhibitors of intracellular signalling affected the FGF7-stimulated shedding of HB-EGF ( Fig. 6e ) or TGFα ( Supplementary Fig. S3c ). The Src-family kinase inhibitors PP2 and Dasatinib significantly reduced constitutive and FGF7-stimulated shedding of HB-EGF and TGFα, whereas the inactive control compound PP3 did not. Moreover, the p38 MAP-kinase inhibitor SB202190 and the PI3-kinase inhibitor LY294002 blocked FGF7-stimulated shedding of HB-EGF and TGFα without significantly reducing its constitutive shedding, whereas the MEK1/2 inhibitor U0126 and the EGFR-selective AG1478 had no significant effect on constitutive or FGF7-stimulated shedding. These results suggest that the activation of ADAM17 by FGFR2b depends on Src, the p38 MAP-kinase and the PI3-kinase, but does not require MEK1/2 or EGFR signalling. Experiments in Src−/− cells rescued with the inactive Src(K295A) or c-Src independently verified that c-Src is required for the FGF7-stimulated shedding of HB-EGF or TGFα from these cells ( Supplementary Fig. S4a,b ). When we tested how the inhibitors that block activation of ADAM17 by FGFR2b affect migration of HaCaT cells, we found that Dasatinib and AG1478 blocked FGF7-stimulated migration, whereas the MEK1/2 inhibitor U0126 did not ( Fig. 7a , a quantification of three separate experiments is shown in Fig. 7b ). The inhibitory effect of Dasatinib could only be partially reversed by addition of HB-EGF, in contrast to the effect of AG1478. Dasatinib weakly inhibited HB-EGF-stimulated migration of HaCaT cells, demonstrating that it also has a direct effect on the EGFR pathway ( Fig. 7a ). Finally, we found that siRNA against AKT, p38 MAP-kinase or Src blocked FGF7-stimulated migration of HaCaT cells ( Fig. 7c ). The block of FGF7-stimulated cell migration by siRNA against AKT or p38 MAP-kinase could be rescued by HB-EGF, whereas the block by siRNA against Src could not ( Fig. 7c , quantification of three separate experiments shown in Fig. 7d ). Separate control experiments corroborated the reduction in the expression of AKT, p38 MAP-kinase and c-Src in HaCaT cells treated with the respective siRNAs ( Fig. 7e–g ). 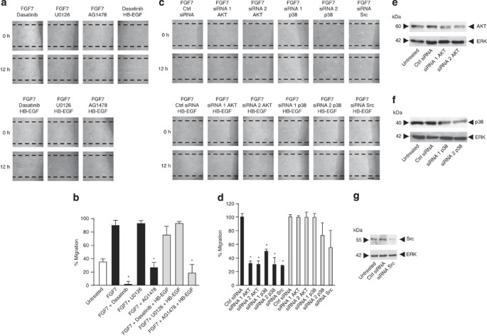Figure 7: Evaluation of the role of various signalling pathways in FGF7-stimulated migration of HaCaT cells. (a) HaCaT cells were treated with or without 50 ng ml−1FGF7 or 50 ng ml−1HB-EGF in the presence or absence of the Src kinase inhibitor Dasatinib (10 μM), the MEK1/2 inhibitor U0126 (10 μM) or the EGFR-kinase inhibitor AG1478 (1 μM). A cell-free area was introduced with a pipette tip, and migration was evaluated after 12 h. One representative example of cells at 0 and 12 h from three independent experiments is shown. Scale bar, 100 μm. (b) Quantification of the results of three separate scratch-wound assays using the inhibitors described ina. (c) In experiments like those described ina, the involvement of AKT, p38 MAP-kinase and Src in FGF7-stimulated HaCaT migration was assessed by transfection with siRNA against these molecules in the presence or absence of HB-EGF. The quantification of three separate experiments is shown ind. Asterisks (*) indicate a significant decrease in scratch wound healing compared with the FGF7-treated samples without inhibitors. Black bars: treated with FGF7, grey bars: treated with FGF7 and HB-EGF. (e–g) Western blot analysis of the expression of AKT (e), p38 MAP-kinase (f) and Src (g) corroborates the reduction in expression of these proteins following treatment with the corresponding siRNAs, as indicated, with a blot for ERK serving as loading control.n=3, ±s.e.m; Student'st-test *P≤0.05. Figure 7: Evaluation of the role of various signalling pathways in FGF7-stimulated migration of HaCaT cells. ( a ) HaCaT cells were treated with or without 50 ng ml −1 FGF7 or 50 ng ml −1 HB-EGF in the presence or absence of the Src kinase inhibitor Dasatinib (10 μM), the MEK1/2 inhibitor U0126 (10 μM) or the EGFR-kinase inhibitor AG1478 (1 μM). A cell-free area was introduced with a pipette tip, and migration was evaluated after 12 h. One representative example of cells at 0 and 12 h from three independent experiments is shown. Scale bar, 100 μm. ( b ) Quantification of the results of three separate scratch-wound assays using the inhibitors described in a . ( c ) In experiments like those described in a , the involvement of AKT, p38 MAP-kinase and Src in FGF7-stimulated HaCaT migration was assessed by transfection with siRNA against these molecules in the presence or absence of HB-EGF. The quantification of three separate experiments is shown in d . Asterisks (*) indicate a significant decrease in scratch wound healing compared with the FGF7-treated samples without inhibitors. Black bars: treated with FGF7, grey bars: treated with FGF7 and HB-EGF. ( e – g ) Western blot analysis of the expression of AKT ( e ), p38 MAP-kinase ( f ) and Src ( g ) corroborates the reduction in expression of these proteins following treatment with the corresponding siRNAs, as indicated, with a blot for ERK serving as loading control. n =3, ±s.e.m; Student's t -test * P ≤0.05. Full size image FGFR2b is shed by ADAM10 Finally, as the shedding of VEGFR2 by ADAM17 is activated by VEGF-A [4] , we wanted to determine whether FGFR2b is itself shed, and if so, identify the responsible sheddase and test whether it responds to stimulation with FGF7. In shedding experiments with FGFR2b in cells lacking ADAM10 or ADAM17 we identified ADAM10 as the principal sheddase for FGFR2b ( Supplementary Fig. S5 ). However, as ADAM10 is not activated by FGFR2b (see above), FGF7 stimulation most likely does not trigger the shedding of FGFR2b itself. Instead, FGFR2 activates ADAM17, leading to the release of HB-EGF and activation of the EGFR/ERK1/2 pathways and cell migration in keratinocytes. The main goal of this study was to probe how the receptor tyrosine kinase FGFR2b activates ERK1/2 signalling and cell migration. Using gain- and loss-of-function studies together with pharmacological inhibitors, we found that stimulation of FGFR2b in primary keratinocytes and HaCaT cells trigger ADAM17-dependent release of EGFR-ligands into the culture supernatants of these cells. Moreover, we demonstrated that a signalling axis that depends on ADAM17>HB-EGF>EGFR is crucial for the activation of cell migration in keratinocytes by FGF7. These results suggest that the well-established role of EGFR in skin homoeostasis and wound healing [31] could also depend on the release of EGFR-ligands by ADAM17, which will be addressed in future studies using conditional knockout mice lacking ADAM17 in the skin. Moreover, the finding that a metalloproteinase and the HB-EGF>EGFR signalling pathway is also necessary for VEGF-A-stimulated migration of HUVEC cells in vitro could help to explain the reduced pathological neovascularization observed in mice lacking the principal HB-EGF sheddase ADAM17 in endothelial cells [32] and the impaired vessel formation in ADAM17-deficient mice [33] . The cross talk between FGFR2b and ERK1/2 is the first example, to our knowledge, of a tyrosine kinase receptor-dependent ERK1/2 phosphorylation that relies entirely on stimulation of ADAM17. By comparison, activation of the VEGFR2 triggers ERK1/2 phosphorylation by at least two mechanisms, the first leading to an initial strong activation of ERK1/2 that is not dependent on ADAM17 and that overshadows the metalloproteinase-dependent component in the first few minutes, and a second that only becomes apparent 15 min after addition of VEGF-A to HUVECs and that involves activation of ADAM17 (ref. 4 ). The activity of the metalloproteinase-dependent component in the first minutes could nevertheless be visualized when the conditioned supernatants from VEGF-A-treated HUVECs were applied to A431 cells, which provided a readout for the presence of soluble EGFR ligands in these supernatants. In these experiments, the time course and MM-sensitivity of ERK1/2 phosphorylation elicited in A431 cells by supernatants from VEGF-A-treated HUVECs was comparable to that triggered by FGF7-stimulated human keratinocytes. In both cases, the metalloproteinase-dependent release of EGFR-ligands into the culture supernatants was activated rapidly, within 5 min of addition of the growth factor. Previous studies have shown that several other activators of keratinocyte migration and/or proliferation, such as PAR1, the angiotensin II type 1 receptor or the anti-microbial peptide Cathelicidin hCAP18/LL-37, also depend on HB-EGF and activation of EGFR [34] , [35] , [36] . As ADAM17 has emerged as the (patho)physiologically relevant sheddase for HB-EGF in cell-based assays and in heart valve development in vivo [13] , [14] , [28] , it is tempting to speculate that these other stimuli of keratinocyte migration also function via an activation of ADAM17. Consistent with this hypothesis, ADAM17 is known to be activated by a variety of distinct stimuli, including thrombin/PAR1 and TNFα [30] , angiotensin II [37] , LPS/Toll-like receptor 4 (ref. 38 ) and G-protein coupled receptors [5] . However, even though ADAM17 is evidently activated by a variety of different signalling pathways, the mechanism underlying its rapid activation by FGF7 and other stimuli remains to be established. Several studies have implicated cytoplasmic phosphorylation of ADAM17 in its activation [29] , [39] , [40] , yet our results suggest that the activation of ADAM17 by FGF7/FGFR2b does not depend on its cytoplasmic domain. Instead, the transmembrane domain of ADAM17 is critical for its ability to respond to stimulation by FGFR2b, which is consistent with the findings of a recent study that analysed the activation of ADAM17 by stimuli such as lysophosphatidic acid, thrombin, TNFα and EGF [30] . Taken together, the results presented here provide evidence for a triple membrane spanning signalling pathway, in which stimulation of the receptor tyrosine kinases FGFR2b or VEGFR2 activates ADAM17, followed by release of HB-EGF and activation of EGFR (see model in Fig. 8 ). Moreover, our results demonstrate that the activation of ADAM17 by FGFR2b depends on Src, PI3-kinase and p38 MAP-kinase. Interestingly, previous studies have shown that Src, which can activate ADAM17 (ref. 41 ), and PI3-kinase are important for FGF7-stimulated keratinocyte migration [42] , suggesting that this also depended on the activation of ADAM17. Thus, ADAM17 has emerged as a critical component of the cross talk between the receptor tyrosine kinases FGFR2b and VEGFR2 and the EGFR/ERK1/2 pathways with a key role in stimulating cell migration elicited by the FGF7/FGFR2b and VEGF-A/VEGFR2 signalling pathways. 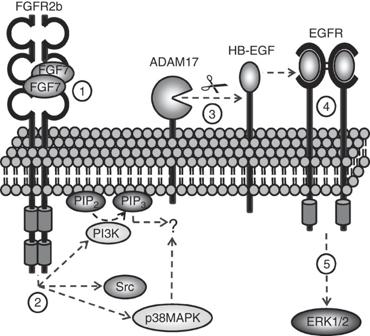Figure 8: A model for transactivation of the EGFR/ERK1/2 signalling pathway by FGF7/FGFR2b. Binding of FGF7 to FGFR2b (1) stimulates ADAM17 in a manner that can be blocked by inhibitors of Src kinases, p38 MAP-kinase and of phosphatidylinositol 3 (PI3) kinase, which is responsible for the conversion of phosphatidylinositol 4,5-bisphosphate (PIP2) to phosphatidylinositol 3,4,5-trisphosphate (PIP3) (2). Stimulation of ADAM17 by FGF7 requires its transmembrane domain, but not the cytoplasmic domain. Activation of ADAM17 triggers release of membrane proteins that include the EGFR-ligand HB-EGF (3), which activates EGFR (4) and ERK1/2 (5), thereby promoting FGF7-stimulated cell migration in keratinocytes. Both FGFR2b and EGFR are known to have critical roles in skin repair and inflammation of the skin21,57. Figure 8: A model for transactivation of the EGFR/ERK1/2 signalling pathway by FGF7/FGFR2b. Binding of FGF7 to FGFR2b (1) stimulates ADAM17 in a manner that can be blocked by inhibitors of Src kinases, p38 MAP-kinase and of phosphatidylinositol 3 (PI3) kinase, which is responsible for the conversion of phosphatidylinositol 4,5-bisphosphate (PIP 2 ) to phosphatidylinositol 3,4,5-trisphosphate (PIP 3 ) (2). Stimulation of ADAM17 by FGF7 requires its transmembrane domain, but not the cytoplasmic domain. Activation of ADAM17 triggers release of membrane proteins that include the EGFR-ligand HB-EGF (3), which activates EGFR (4) and ERK1/2 (5), thereby promoting FGF7-stimulated cell migration in keratinocytes. Both FGFR2b and EGFR are known to have critical roles in skin repair and inflammation of the skin [21] , [57] . Full size image Primary cells and cell lines Cos-7 cells were from ATCC. HUVECs (provided by S.R.) were cultured on gelatin-coated plates in EC medium: M199 (Bio-Whittaker), 20% fetal bovine serum, 90 U ml −1 heparin and 20 ng ml −1 endothelial growth factor supplement (Sigma). The human keratinocyte line HaCaT [43] was from N. Fusenig (Deutsches Krebsforschungszentrum, Heidelberg, Germany). Adam10−/− mEFs were from Dr Paul Saftig (University of Kiel, Kiel, Germany), Src−/− mEFs were from Dr Xin-Yun Huang (Cornell University, New York) and Adam17 −/− mEFs were from CB's lab [38] , [44] , [45] . Primary human foreskin keratinocytes (PromoCell) were cultured in keratinocyte growth medium-2 (KGM-2; PromoCell). Primary mouse keratinocytes were isolated and cultured in KGM-2 supplemented with 20 ng ml −1 murine EGF and 8 ng ml −1 Cholera toxin (Sigma). To generate ADAM17-deficient primary keratinocytes, B6.Cg-Tg(CAG-cre/Esr1*)5Amc/J mice containing a Tamoxifen-inducible Cre expressed under the control of the chicken beta actin promoter/enhancer (Jackson Labs, referred to as CAG-Cre throughout) were crossed with mice carrying floxed alleles of ADAM17 (ref. 38 ). The littermate-offspring of matings between Adam17flox/flox/CAG-Cre and Adam17flox/flox mice were used for isolation of primary keratinocytes as follows: 12-week-old mice were euthanized, and their tail was removed and disinfected for 5 min in Triadine (Triad Disposables). After washing in 70% ethanol the skin was removed and cut into small pieces, which were spread dermal side down on sterile Whatman paper and incubated in serum-free DMEM with 1% trypsin for 90 min at 37 °C. The epidermis was separated from the dermis, transferred to PBS, 10% FCS and the resulting cell suspension was passed through a 40 μm cell-filter and centrifuged for 5 min at 200 g . The sedimented cells were resuspended in KGM-2, seeded in Collagen-coated six-well plates (Becton-Dickinson) and used at a confluence of 80–90%. The medium was changed every second day. All animal experiments were approved by the Internal Animal Use and Care Committee of the Hospital for Special Surgery. All other cell lines were grown in DMEM supplemented with antibiotics and 5% FCS. Growth factors and inhibitors Recombinant human heparin-binding EGF (HB-EGF), Thrombin, Human vascular endothelial growth factor (VEGF-A), Murine epidermal growth factor (EGF), and murine and human Fibroblast Growth Factor 7 (FGF7, also referred to as keratinocyte growth factor) were from R&D Systems. PMA (phorbol-12-myristate-13-acetate), the EGFR tyrosine kinase inhibitor Thyrphostin (AG1478) and the mutant diphtheria toxin CRM197 were from Sigma. The MEK1/2 inhibitor U0126, the p38 MAP-kinase inhibitor SB202190, the Phosphatidylinositol 3-kinase inhibitor LY294002, the Calcium ionophore, Ionomycin and the Src-family kinase inhibitor PP2 and its inactive analogue PP3 were from EMD Chemicals. Dasatinib was from Mark Moasser. The metalloproteinase inhibitor MM was from Ouathek Ouerfelli, Sloan-Kettering Institute, New York, New York [46] . The EGFR-function blocking antibody Cetuximab (C225) was from Merck. Antibodies Rabbit anti-phospho ERK1/2, anti-phospho FRS2, anti-phospho EGFR, anti-EGFR, anti-Src and anti-AKT were from Cell Signaling Technology. Rabbit anti-ERK2, >anti-p38 and anti-GAPDH were from Santa Cruz Biotechnology. Anti-FGFR2 antibodies were from Sigma and Anti-HA antibodies from Covance. Rabbit polyclonal anti-ADAM17 cytotail antibodies were from CB's laboratory [47] . Expression vectors The expression vectors for ADAM10 and ADAM10E>A were from Dr Paul Saftig [48] , for ADAM17 from Dr Gillian Murphy (University of Cambridge, UK). The expression constructs for ADAM17E>A, ADAM17Δ–cyto, ADAM17-CD62L [27] , [30] , [49] , full-length and AP-tagged FGFR2b [50] , [51] , AP-tagged CD40 (ref. 4 ), TNFα [52] and TGFα [14] were from CB's laboratory. Transfection and ectodomain shedding assay Fibroblasts and HaCaTs were transfected with Lipofectamine2000, and Cos-7 cells were transfected with Lipofectamine [14] , [53] . For shedding experiments (performed one day after transfection), cells were washed with OptiMEM, which was replaced after 1 h by fresh OptiMEM with or without the indicated inhibitors or stimuli, and then incubated for 30 min to 4 h (ref. 14 ). The AP activity in the supernatant and cell lysates was measured at A405 after incubation with the AP substrate 4-nitrophenyl phosphate [14] , [54] . No AP activity was present in conditioned media of non-transfected cells. Three identical wells were prepared, and the ratio between the AP activity in the supernatant and the cell lysate plus supernatant were calculated for normalization. Each experiment was performed in three tissue culture wells, and repeated at least three times. Small interfering RNA transfection For silencing of ADAM17, HaCaTs were grown to 40–50% confluency and transfected with 2 μl Stealth Small Interfering RNA (siRNA) duplex (HSS186-181, Invitrogen) using Lipofectamine 2000. For silencing of AKT, p38 MAP-kinase or Src, HaCaTs were grown to 40–50% confluency and transfected with 50 nM Stealth siRNA duplex (#6211, #6510, #6564, #6243 or #6568, Cell Signaling Technology or sc-29228 Santa Cruz Biotechnology) using TransIT-TKO (Mirus). Random Stealth siRNA duplexes coding for non-functional RNAs served as controls. After 60 h incubation at 37 °C, the cells were starved in Opti-MEM for 8 h and used in scratch wound assays. Afterwards the cells were processed for western blot analysis to analyze knockdown efficiency. Western blot analysis Cells were lysed on ice in Tris-buffered saline (TBS) Triton-X100 (1%), 1 mM EDTA, 1,10-Phenanthroline (10 mM), Protease inhibitor cocktail and Phosphatase-inhibitor (Roche Applied Science). Comparable amounts of protein were separated on 10% SDS-polyacrylamide gels, and transferred onto polyvinylidene difluoride membranes (BioTrace, Pall Corporation). These were blocked with 3% skim milk in TBS, then incubated with primary antibodies, washed in 0.1% Tween-TBS and bound primary antibodies were detected with Peroxidase-conjugated goat anti-mouse or goat anti-rabbit antibodies (Promega) using the ECL detection system (Amersham Biosciences) and a Chemdoc image analyzer (BioRad). To generate the control blots for expression of ERK1/2, separate western blots were prepared and probed as indicated, with the exception of the control blots in Figures 2 , 3e , 4g and 5c,e,g and Supplementary Figures S1c and S2c , which were incubated in stripping reagent (100 mM 2-mercaptoethanol, 2% (w/v) SDS, 62.5 mM Tris-HCL pH 6.7) at 55 °C for 30 min and then re-probed with anti ERK1/2 antibody. In vitro scratch wound-healing assays All cells used for in vitro scratch wound-healing assays (primary mouse or human keratinocytes, HaCaTs or HUVECs) were seeded in 12-well plates and cultured until they reached confluence. A scratch wound was introduced with a 200 μl pipette tip. After washing with PBS the cells were incubated with or without the indicated inhibitors or stimuli. After different periods of time, cells at the same positions along the scratch wound (marked with an indelible marker) were photographed using an Inverted phase-contrast microscope (Nikon, Eclipse TS100), and NIH Image J software was used for quantification of scratch wound assays [55] . Cell proliferation assay Primary mouse keratinocytes from Adam17flox/flox control mice or Adam17flox/flox/CAG-Cre mice were treated with or without 1 μM Tamoxifen for 48 h and then seeded at 2×10 4 cells per well in 96-well plates. After 1 day, cells were treated with FGF7, HB-EGF or left untreated. The media was removed after 72 h and replenished with fresh, untreated media and a MTS [3-(4,5-dimethyl-2-yl)-5-(3 carboxymethoxyphinyl)-2-(4-sulphophenyl)-2H-tetrazolium] assay was performed following the manufacturer's instructions (Promega). EGFR ligand release assay Primary human keratinocytes or HUVECs on 6-well plates were treated with either FGF7 or VEGF-A, respectively, and incubated in the presence or absence of different inhibitors for 5–60 min in Optimem medium. Conditioned supernatants (500 μl) were removed and incubated for 10 min with A431 cells, which express high levels of EGFR/ErbB1 (ref. 56 ). The A431 cells were serum-starved overnight before the addition of the conditioned supernatants. For the experiments with AG1478 (1 μM) or the EGFR-blocking antibody Cetuximab (10 μg ml −1 ), these compounds were pre-incubated with A431 cells for 10 min in Optimem before adding the conditioned media from stimulated cells, which was adjusted to 1 μM AG1478 or 10 μg ml −1 Cetuximab as indicated. All conditioned supernatants were adjusted to the same concentration of MM (5 μM) before addition to A431 cells to control for effects of this metalloproteinase inhibitor on A431 cells. Statistical analysis All values are expressed as means±standard error of the mean. The standard error values indicate the variation between mean values obtained from at least three independent experiments. Statistics following a Student t distribution were generated using the t -test. P values of <0.05 were considered as statistically significant. How to cite this article: Maretzky, T. et al . Migration of growth factor-stimulated epithelial and endothelial cells depends on EGFR transactivation by ADAM17. Nat. Commun. 2:229 doi: 10.1038/ncomms1232 (2011).